Concurrent transition of ferroelectric and magnetic ordering near room temperature Strong spin-lattice coupling in condensed matter gives rise to intriguing physical phenomena such as colossal magnetoresistance and giant magnetoelectric effects. The phenomenological hallmark of such a strong spin-lattice coupling is the manifestation of a large anomaly in the crystal structure at the magnetic transition temperature. Here we report that the magnetic Néel temperature of the multiferroic compound BiFeO 3 is suppressed to around room temperature by heteroepitaxial misfit strain. Remarkably, the ferroelectric state undergoes a first-order transition to another ferroelectric state simultaneously with the magnetic transition temperature. Our findings provide a unique example of a concurrent magnetic and ferroelectric transition at the same temperature among proper ferroelectrics, taking a step toward room temperature magnetoelectric applications. Multiferroics, where ferroelectricity and magnetism coexist, have inspired physicists to address the delicate interplay of spin and lattice degrees of freedom [1] , [2] , [3] , [4] , [5] , [6] , [7] , [8] , [9] , [10] . Bismuth ferrite, BiFeO 3 (BFO), has been in a particular position in multiferroic studies. It is one of the most promising magnetoelectric materials because of the exceptionally large order parameters—both magnetic and electric—at room temperature. Moreover strong magnetoelectric effect of the BFO has been explored in the form of voltage-driven flipping of the magnetic plane [11] , [12] . Recently it has been reported that a highly elongated phase of BFO in a tetragonal-like form (c.a. ~1.26) can be stabilized through heteroepitaxial misfit strain by coherent growth on LaAlO 3 substrates [13] , [14] . It has been observed that normal BFO (R-BFO) and the highly elongated tetragonal-like BFO (T-BFO) are both switchable by electric field, producing a colossal electrostrain as a result of the two-phase competition [14] . The bulk phase of R-BFO has a rhombohedral symmetry (space group: R 3c) with large remanent polarization of ~90 μC cm −2 . Its ferroelectric Curie temperature is ~1103 K and the G-type antiferromagnetic Néel temperature T N is ~640 K with a long periodic cycloidal spiral spin arrangement [15] , [16] , [17] . The effect of strain on the T N of R-BFO films has been systematically examined [18] . However, physical properties of T-BFO remains less explored except for some theoretical and Raman spectroscopic studies [19] , [20] , [21] , [22] , ferroelectric domain and crystal structure at room temperature [23] , [24] , [25] , and very recently published temperature-driven structural phase transition [26] , [27] . In this paper, we report that the magnetic Néel temperature of the T-BFO is largely decreased to near room temperature. Possible mechanisms to suppress the magnetic order will be discussed on the basis of experimental evidence of a peculiar bonding character. In addition, we show that the ferroelectric state abruptly changes at T N , providing a unique example to show the concurrent transition of the magnetic order and ferroelectric state among proper ferroelectrics. Finally we will report intriguing magnetoelectric properties of the T-BFO around the transition temperature. Determination of magnetic transition temperature First, we focus on the magnetic transition temperature of the highly elongated BFO phase. To clarify the magnetic order, we employed the magnetic linear dichroism (MLD) in the Fe L -edge X-ray absorption spectroscopy (XAS) [28] . This technique offers a powerful tool to explore the antiferromagnetic order of the thin layer in an element-specific way. 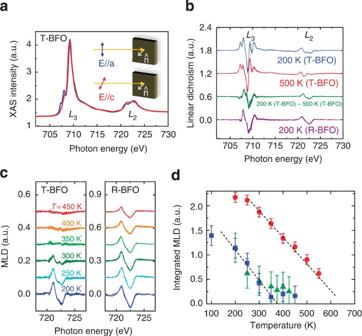Figure 1: Determination ofTNfrom FeL2,3-edge X-ray magnetic linear dichroism (XMLD) of T-BFO and R-BFO films. (a) FeL2,3-edge X-ray absorption spectra of T-BFO for different polarizations (E//aand E//c). (b) LD spectra (E//a–E//c) of T-BFO at 200 and 500 K, and MLD spectrum obtained by subtracting the 500 K LD spectrum, which gives only the o-LD term, in comparison with the LD spectrum of R-BFO at 200 K, which is regarded as the MLD one. The obtained MLD spectrum of T-BFO agrees well with that of R-BFO, which shows the typical MLD line shape of a ferrite with Fe3+. (c) FeL2edge XMLD spectra of T-BFO and R-BFO films at different temperatures. (d) Integrated MLD intensity (IMLD), which is proportional to the square of the magnetic order parameter, as a function of temperature. Circle symbols represent the IMLDof a R-BFO film; square and triangular symbols represent the IMLDof two independent T-BFO1and T-BFO2films, respectively. IMLDfollows the linear dashed line nearTNfor R-BFO and T-BFO, which is determined to be ~640 and ~380 K, respectively. The error bars were determined by the maximum deviation in separate analyses. The XAS spectra are divided into the L 3 (2 p 3/2 ) and L 2 (2 p 1/2 ) regions due to the large 2 p core hole spin-orbit coupling energy, as shown in Figure 1a . The spectra strongly depend on the photon polarization, which is parallel (E|| a ) or perpendicular (E|| c ) to the in-plane crystalline axis of the film, and yield large linear dichroism by subtracting the E|| c spectrum from the E|| a one. Particularly in antiferromagnetic materials with strong structural anisotropy, the linear dichroism (LD) has contributions from both the orbital and magnetic anisotropy. In most ferroic perovskites with the half-filled Fe 3+ (3 d 5 ) ion at the centre of the regular (or slightly tilted) oxygen octahedron, the orbital anisotropy (involving the structural anisotropy) is minimal, and the LD is dominated by the magnetic anisotropy. The normal R-BFO belongs to this case, even though the Fe ions are shifted to an off-centered position. In the T-BFO, however, the octahedron is so strongly elongated along the c -axis (c.a.~1.26) that the LD is also strongly affected by the contribution due to the orbital anisotropy. Thus to obtain the magnetic ordering information rigorously, it is necessary to separate the MLD signal from the LD signal strongly mixed by the magnetic and orbital contributions. Figure 1: Determination of T N from Fe L 2,3 -edge X-ray magnetic linear dichroism (XMLD) of T-BFO and R-BFO films. ( a ) Fe L 2,3 -edge X-ray absorption spectra of T-BFO for different polarizations (E// a and E// c ). ( b ) LD spectra (E// a –E// c ) of T-BFO at 200 and 500 K, and MLD spectrum obtained by subtracting the 500 K LD spectrum, which gives only the o-LD term, in comparison with the LD spectrum of R-BFO at 200 K, which is regarded as the MLD one. The obtained MLD spectrum of T-BFO agrees well with that of R-BFO, which shows the typical MLD line shape of a ferrite with Fe 3+ . ( c ) Fe L 2 edge XMLD spectra of T-BFO and R-BFO films at different temperatures. ( d ) Integrated MLD intensity (I MLD ), which is proportional to the square of the magnetic order parameter, as a function of temperature. Circle symbols represent the I MLD of a R-BFO film; square and triangular symbols represent the I MLD of two independent T-BFO 1 and T-BFO 2 films, respectively. I MLD follows the linear dashed line near T N for R-BFO and T-BFO, which is determined to be ~640 and ~380 K, respectively. The error bars were determined by the maximum deviation in separate analyses. Full size image In the following we introduce our strategy to subdivide LD into the orbital and magnetic contributions. The MLD originates from the antiferromagnetic order and thus depends on temperature significantly near T N —it decreases continuously with the magnetic order parameter and vanishes above T N . On the other hand, the orbital LD (o-LD) is basically attributed to the Fe 3 d orbital level splitting involving the anisotropic structure distortion. As the level splitting are of the order of a few hundred meV as discussed below, the o-LD is not expected to vary severely with temperature in the range of the measurement. Indeed, we found that the LD line shape shows significant temperature dependence below 400 K in T-BFO but barely varies with temperature above reflecting the nearly temperature-independent o-LD contribution. Thus we are able to extract MLD from the mixed LD subtracting out the o-LD term (we adopted the LD spectrum at 500 K as the o-LD one, but the result does not change even when we choose another LD one at 400 or 450 K). Figure 1b shows the representative LD spectra of T-BFO at 200 K before and after subtraction of the o-LD term (the 500 K LD spectrum) in comparison with the LD spectrum of R-BFO. One can easily recognize that the subtracted LD one shows a line shape nearly identical to the LD one of R-BFO, which displays a typical MLD line shape pattern, a positive left half and a negative right half, as reported previously [28] . With this correction, we could obtain the reliable MLD spectra of T-BFO for various temperatures ( Fig. 1c ). We confirmed nearly the same results in two independent measurements. By using the integration of the MLD intensity for different temperatures, (which corresponds to the square of the magnetic order parameter) we successfully determined that T N ≈380 K for the T-BFO, which is much lower than T N ≈640 K of R-BFO ( Fig. 1d ). This is intuitively understandable given the large structural anisotropy of this phase as discussed below. Moreover, the systematic configuration interaction model calculations including the full atomic multiplets and crystal field splitting exactly reproduce the fine structures of the LD line shape above and below T N ( Supplementary Fig. S1 and Supplementary Note 1 ). Spectroscopic evidence of oxygen pyramidal structure To understand why the highly elongated phase has the abnormally large dichroism arising from the orbital anisotropy and why the Néel temperature is largely suppressed to near room temperature, the electronic state of the 3 d levels should be clarified (note that such a large change in T N by strain is not a common phenomenon). 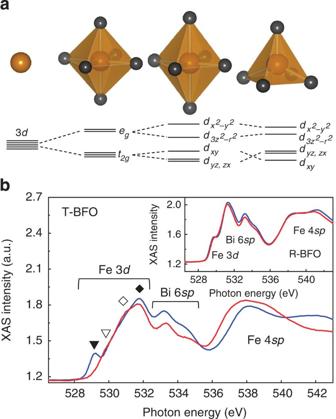Figure 2: Fe 3dlevel splits and OK-edge X-ray absorption spectra of T-BFO. (a) Schematic representation of the transition metal oxide local structures and the 3dlevel splits in the spherical, octahedral (Oh), elongated tetragonal (D4h) and square pyramidal (C4v) site symmetries. In the highly elongated tetragonal case, the transition metal ion shifts along an apical direction for relief of the large Coulomb repulsion energy. This metal shift brings on thedxyanddyz/dzxenergy level switching. (b) OxygenK-edge absorption spectra for different polarizations (E//a(blue line) and E//c(red line)) of T-BFO and R-BFO. The spectra, reflecting the conduction band, are roughly divided into three regions, Fe 3d, Bi 6spand Fe 4spstates hybridized with O 2pstates. In the T-BFO case, the spectrum exhibits large polarization dependence induced by the strong orbital anisotropy. Thedxyorbital state (indicated by the filled triangle)dyz/dzx(empty triangle),dx2−y2(filled diamond) andd3z2-r2(empty diamond) were identified in the strict dipole selection rule. (Inset) In the R-BFO case, the spectrum shows very small polarization dependence resulting from the weak orbital anisotropy. Figure 2a displays a schematic representation of transition metal oxide local structures and site symmetries. According to the ligand field theory, the fivefold degenerated 3 d level is split into triplet t 2g and doublet e g levels in the octahedral (O h ) symmetry. The elongation of the octahedron along the c -axis reduces to the tetragonal (D 4h ) symmetry and generates additional Jahn–Teller-type level splitting [29] . In the T-BFO phase, the elongation is extremely large and is accompanied with a large Fe shift along the c -axis to relieve the strong Coulombic repulsion between the Fe ion and neighbouring oxygen ions in the ab plane. As a result, the local structure becomes the FeO 5 pyramid in the C 4v site symmetry, where the in-plane xy orbital level becomes the lowest. This cation-shifted oxygen pyramidal structure is exactly what happens in the highly elongated T-BFO phase. Figure 2: Fe 3 d level splits and O K -edge X-ray absorption spectra of T-BFO. ( a ) Schematic representation of the transition metal oxide local structures and the 3 d level splits in the spherical, octahedral (O h ), elongated tetragonal (D 4h ) and square pyramidal (C 4v ) site symmetries. In the highly elongated tetragonal case, the transition metal ion shifts along an apical direction for relief of the large Coulomb repulsion energy. This metal shift brings on the d xy and d yz / d zx energy level switching. ( b ) Oxygen K -edge absorption spectra for different polarizations (E// a (blue line) and E// c (red line)) of T-BFO and R-BFO. The spectra, reflecting the conduction band, are roughly divided into three regions, Fe 3 d , Bi 6 sp and Fe 4 sp states hybridized with O 2 p states. In the T-BFO case, the spectrum exhibits large polarization dependence induced by the strong orbital anisotropy. The d xy orbital state (indicated by the filled triangle) d yz / d zx (empty triangle), d x2−y2 (filled diamond) and d 3z2-r2 (empty diamond) were identified in the strict dipole selection rule. (Inset) In the R-BFO case, the spectrum shows very small polarization dependence resulting from the weak orbital anisotropy. Full size image Experimental evidence of the pyramidal C 4v symmetry can be confirmed in the polarization-dependent O K -edge XAS, which directly shows transferred O 2 p partial density due to hybridization with the unoccupied orbital states [30] . As seen in Figure 2b , the spectra are roughly divided into Fe 3 d , Bi 6 sp and Fe 4 sp orbital character regions for both R-BFO and T-BFO. In R-BFO, the spectrum does not vary much for the different incoming photon polarization (E|| c and E|| a ) indicating that the orbital anisotropy is relatively small. It is also consistent with the fact that the o-LD term is negligible and the Fe L -edge LD of R-BFO is regarded as MLD, as discussed previously. In contrast, the O K -edge spectrum of T-BFO exhibits strong polarization dependence, particularly in the Fe 3 d region, reflecting the strong orbital anisotropy, as also observed in the Fe L -edge LD. Taking advantages of the strict dipole selection rules in the polarization-dependent XAS (the E|| c light enhances the absorption to the O 2 p states hybridized with the out-of-plane d yz/zx and d 3 z 2− r2 orbitals whereas the E ⊥ c light does one to the O 2 p states hybridized with the in-plane d xy and d x2−y2 orbitals), we can confidently identify the four distinguishable Fe 3 d orbital states in the conduction band as indicated in Figure 2b . The identified 3 d orbital level splitting exactly coincides with those in the pyramidal C 4v symmetry, including the lowest energy d xy orbital state, whereas they are against the elongated tetragonal D 4h level splitting. These results experimentally provide strong spectroscopic evidence on the formation of the FeO 5 pyramid resulting from the highly off-centered Fe position in T-BFO. We now turn to the discussion of the suppression of the magnetic Néel temperature in T-BFO. BFO is expected to have strong G-type anti-ferromagnetic ordering because the half-filled d 5 electron configuration leads to a strong anti-ferromagnetic super-exchange interaction between all nearest neighbouring Fe 3+ ions [29] . As expected, the Néel temperature of the R-BFO is very high at 640 K, which is comparable to that of other perovskite rare-earth ferrites ( R FeO 3 ) [31] , [32] . On the other hand, the Néel order of T-BFO is strongly suppressed. The strength of exchange interaction ( J ), which directly controls the Néel temperature, is estimated to be J ≈| t pd | 4 / U / Δ 2 , where t pd stands for an overlap integral between Fe d orbital and oxygen 2 p orbital in a one electron Hamiltonian, and U and Δ represent on-site Coulomb repulsion and charge transfer energy, respectively [33] . For d 5 systems, the primary interaction is between two filled e g orbitals through oxygen 2 p σ-bonding. The suppression of antiferromagnetic order is attributed to the decrease of the hopping integral either due to the large Fe-O distance along the c-direction or due to the larger deviations from 180 o of the Fe-O-Fe bond angle within the ab -plane. Structural and dielectric anomaly at the T N With this background of the magnetic and electronic structure, we move on to the structural and dielectric properties of the highly elongated T-BFO phase. Here we report that the T-BFO undergoes large structural and ferroelectric transitions at the magnetic Néel temperature. To characterize the structural properties, we carried out X-ray diffraction using a four-circle X-ray diffractometer. By collecting the position of the (002) c peak in conventional θ-2θ scans and varying temperature, the c -axis lattice parameter of the film was investigated ( Fig. 3a ). Remarkably, the c -axis lattice parameter changes abruptly around 380 K with a thermal hysteresis of ~25 K. The lattice parameter is changed by ~0.2%, which is a very large value comparable with those of giant magnetostrictive materials such as rare earth alloys [34] , [35] . Furthermore, it is significantly larger than hexagonal manganites (~0.02%) where a giant magnetoelastic coupling has been reported [36] . Besides the sharp hysteresis in the T N , a large range of temperatures where the lattice parameters do not match was also observed. It is probably due to phase coexistence as discussed by Kreisel et al . [26] ; however, we cannot rule out possibility of different strain state of the higher temperature phase according to thermal history. The dielectric properties also have an anomaly at the transition temperature. 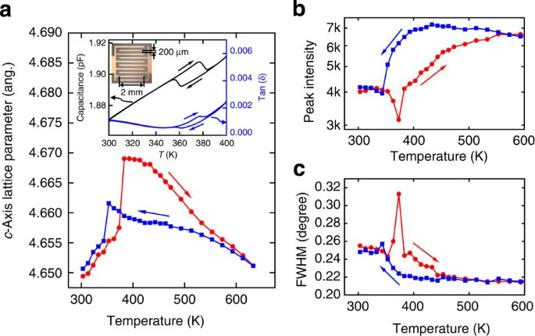Figure 3: Structural and dielectric anomaly at the magnetic Néel temperature. (a) Thec-axis lattice parameter is plotted as a function of temperature. The lattice parameters can be obtained from the position of the (002)cpeaks in X-ray diffraction. At ~380 K, an abrupt change of thec-axis lattice parameter has been observed with a thermal hysteresis of ~25 K, indicating that a first-order structural transition occurs concurrently at the magnetic Néel temperature. (Inset) Capacitance and loss tangent were measured using the displayed interdigitated electrodes as a function of temperature, which also shows a clear first-order transition. (b) The intensity of the (002)cpeak is presented. The structural phase at the higher temperature has stronger peak intensity. (c) The full-width-at-half-maximum (FWHM) of the (002)cpeak is presented. As shown in the inset of Figure 3a , clear thermal hysteresis in the capacitance and the loss tangent indicate the transition is of first-order type, reflecting a competing nature of the two structural phases. The transition can be repeatedly observed during many cycles of heating and cooling and it was repeatable in multiple samples. The higher temperature phase has a larger c -axis lattice parameter and the peak intensity of the (002) c peak becomes stronger ( Fig. 3b ). Around the transition temperature, the full-width-at-half-maximum of the peak is increased ( Fig. 3c ). Such a structural anomaly at the magnetic transition temperature has never been observed in normal R-BFO ( Supplementary Fig. S2 and Supplementary Note 2 ). Figure 3: Structural and dielectric anomaly at the magnetic Néel temperature. ( a ) The c -axis lattice parameter is plotted as a function of temperature. The lattice parameters can be obtained from the position of the (002) c peaks in X-ray diffraction. At ~380 K, an abrupt change of the c -axis lattice parameter has been observed with a thermal hysteresis of ~25 K, indicating that a first-order structural transition occurs concurrently at the magnetic Néel temperature. (Inset) Capacitance and loss tangent were measured using the displayed interdigitated electrodes as a function of temperature, which also shows a clear first-order transition. ( b ) The intensity of the (002) c peak is presented. The structural phase at the higher temperature has stronger peak intensity. ( c ) The full-width-at-half-maximum (FWHM) of the (002) c peak is presented. 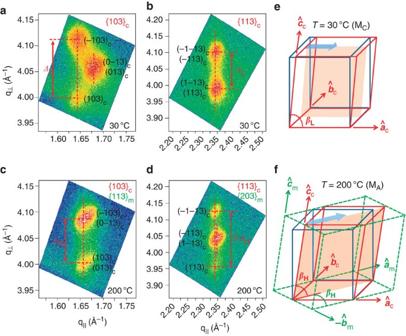Figure 4: Crystal structures characterized by X-ray reciprocal space maps. (a) Reciprocal space map for pseudocubic {103}cpeaks at a representative lower temperature (30°C). (b) Reciprocal space map for {113}cpeaks at 30°C. (c) Reciprocal space mapping for pseudocubic {103}cpeaks was performed at 200°C. (d) Reciprocal space map for {113}cpeaks at 200°C. (e) The pseudocubic unit cell of the lower temperature phase has a monoclinic distortion where thec-axis direction tilts up toward [100]c. The lattice parameters for the pseudocubic unit cell at 30 K areac=3.82(1) Å,bc=3.74(0) Å,cc=4.64(9) Å andβL=88.01°. (f) The pseudocubic unit cell at the higher temperature is presented. In this case, the direction of thec-axis tilt is toward [110]c. The pseudocubic lattice parameters areac≈3.79(3) Å,bc˜3.79(3) Å,cc=4.66(5) Å andβH=87.93°. The dashed line represents more rigorous monoclinic cell, which has a volume of ~√2a×~√2a×c. The lattice parameters of the monoclinic unit cell correspond toam=5.36(3) Å,bm=5.35(3) Å,cm=4.66(5) Å andβH=87.93°. The high temperature structural phase is similar to the normal R-BFO film in terms of the direction of the distortion, however, it is apparently different in terms of the largec-axis lattice parameter. Full size image Crystal structures Detailed crystal structural analyses below and above the transition temperatures were carried out by X-ray reciprocal space mapping as presented in Figure 4a–d . From the peak splitting of the peudocubic (103) c and (113) c reflections, we have discovered that the structural transition corresponds to a monoclinic to monoclinic transition. The lower temperature phase has equal amount of peak splitting in the (103) c and (113) c peaks, whereas the higher temperature phase has a twice larger splitting of the (113) c peaks as compared with the (103) c peaks. The characteristics of the splits are related to the tilt angle and the tilt direction of the monoclinic unit cells. The proposed pseudocubic cells with quantitative lattice parameters are presented in Figure 4e,f (see also Supplementary Figs S3 and S4 , and Methods for the description of how to analyze reciprocal space maps). These monoclinic structures correspond to type of M C (for the low temperature phase) and type of M A (for the high temperature one), according to the notation of Vanderbilt and Cohen [37] . The crystal structure at the low temperature is consistent with the previous results [23] , [24] . These two monoclinic unit cells are highly elongated along the c direction. However, they differ from each other in terms of the monoclinic tilt direction. Interestingly, the mirror plane of the monoclinic unit cell rotates by 45°. Assuming that the ferroelectric polarization lies inside the mirror plane (Point group: m), we can expect that the in-plane component of polarization directs toward [100] c at lower temperature but it will be switched to [110] c at higher temperature. Considering a head-to-tail structure of ferroelectric domains minimizing electrostatic energy at the domain walls, we expect a rotation of ferroelectric stripe domain walls by 45°. Figure 4: Crystal structures characterized by X-ray reciprocal space maps. ( a ) Reciprocal space map for pseudocubic {103} c peaks at a representative lower temperature (30°C). ( b ) Reciprocal space map for {113} c peaks at 30°C. ( c ) Reciprocal space mapping for pseudocubic {103} c peaks was performed at 200°C. ( d ) Reciprocal space map for {113} c peaks at 200°C. ( e ) The pseudocubic unit cell of the lower temperature phase has a monoclinic distortion where the c -axis direction tilts up toward [100] c . The lattice parameters for the pseudocubic unit cell at 30 K are a c =3.82(1) Å, b c =3.74(0) Å, c c =4.64(9) Å and β L =88.01°. ( f ) The pseudocubic unit cell at the higher temperature is presented. In this case, the direction of the c -axis tilt is toward [110] c . The pseudocubic lattice parameters are a c ≈3.79(3) Å, b c ˜3.79(3) Å, c c =4.66(5) Å and β H =87.93°. The dashed line represents more rigorous monoclinic cell, which has a volume of ~√2a×~√2a×c. The lattice parameters of the monoclinic unit cell correspond to a m =5.36(3) Å, b m =5.35(3) Å, c m =4.66(5) Å and β H =87.93°. The high temperature structural phase is similar to the normal R-BFO film in terms of the direction of the distortion, however, it is apparently different in terms of the large c -axis lattice parameter. 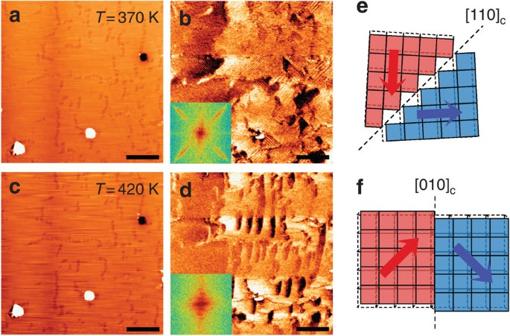Figure 5: Piezoresponse force microscopy below and above the phase transition temperature. (a) Surface morphology of a T-BFO film obtained at a representative low temperature (370 K). (b) Ferroelectric domain image was simultaneously measured with the surface morphology using in-plane PFM. The Fourier transform of the in-plane PFM image is shown in the inset. (c) Surface morphology of the same area was measured at a representative high temperature (420 K). (d) In-plane ferroelectric domain image at 420 K. Ferroelectric domains align along < 100> >cwith wider domain width. The Fourier transformed image is shown in the inset. Scale bars ina,b,canddindicate 2 μm. (e) Schematic illustration represents a ferroelectric domain wall aligned along <110>cat the low temperature. (f) The schematic displays a domain wall at the high temperature. Ineandf, the in-plane polarizations compatible to the monoclinic structural distortions are schematized with domain walls. The direction of out-of-plane polarization is downwards (not shown here). Full size image Ferroelectric domain structures To check the domain structure, we performed in situ piezoresponse force microscopy (PFM) of the same region above and below the transition temperature as shown in Figure 5a–d . As predicted from the crystallographic information, the ferroelectric domain structure does rotate by 45° in the stripe pattern. The phase at lower temperature has dense stripe domains with a typical domain width of ~50 nm along <110> c direction, which is consistent with the PFM images reported by Chen et al . [23] , [25] ; whereas the higher temperature phase has much larger stripe domains, which are elongated along <100> c . This suggests that the domain walls at the higher temperature have a higher energy cost to be stabilized. Regarding elastic deformation at the domain walls ( Fig. 5e,f ), the high temperature phase is probably more unstable because the upper-layer atoms at the domain walls prefer to ferroelastically move along the domain wall but the preferred direction of the shift is exactly opposite with respect to the associated domains. More rigorous studies are needed to gain a complete understanding of this effect. The high temperature domain pattern returns back to the low temperature one reversibly when we cool down to room temperature. The morphologies measured simultaneously along with the PFM images make sure that the measured region did not change under the temperature variation. Figure 5: Piezoresponse force microscopy below and above the phase transition temperature. ( a ) Surface morphology of a T-BFO film obtained at a representative low temperature (370 K). ( b ) Ferroelectric domain image was simultaneously measured with the surface morphology using in-plane PFM. The Fourier transform of the in-plane PFM image is shown in the inset. ( c ) Surface morphology of the same area was measured at a representative high temperature (420 K). ( d ) In-plane ferroelectric domain image at 420 K. Ferroelectric domains align along < 100> > c with wider domain width. The Fourier transformed image is shown in the inset. Scale bars in a , b , c and d indicate 2 μm. ( e ) Schematic illustration represents a ferroelectric domain wall aligned along <110> c at the low temperature. ( f ) The schematic displays a domain wall at the high temperature. In e and f , the in-plane polarizations compatible to the monoclinic structural distortions are schematized with domain walls. The direction of out-of-plane polarization is downwards (not shown here). 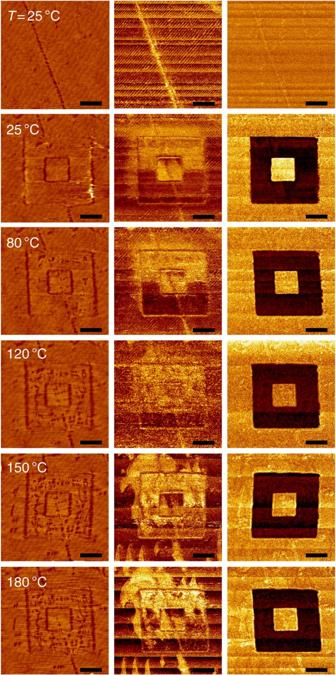Figure 6: Temperature-dependent PFM images of a T-BFO thin film. Three images (surface morphology at the left column, in-plane PFM at the middle column, out-of-plane PFM at the right column) have been taken simultaneously. The measurement sequence is from the top to the bottom, that is, increasing the temperature of the sample. Scale bars represent 1 μm. The PFM images were taken under amplitude contrast. Full size image To further understand temperature effect on the ferroelectric domain structure, we have measured PFM images for a poled region at selected temperatures with heating the film across the Néel temperature as shown in Figure 6 . First of all, we have taken surface morphology, in-plane PFM, and out-of-plane PFM images at a time for the virgin area of T-BFO film grown on Pr 0.5 Ca 0.5 MnO 3 (PCMO)/LaAlO 3 (001) substrate at room temperature (top row in the Fig. 6 ). Fine stripe domain structure along <110> c , a typical domain pattern for the M C phase of T-BFO, has been detected. At room temperature, we applied a poling voltage of −12 V over a 3×3 μm 2 area and then partially poled it back with +12 V on a 1×1 μm 2 area. As a result, we can get clear contrast in the out-of-plane PFM images; the dark area in the out-of-plane PFM image indicates an area with polarization pointing up and the bright area has the polarization pointing down. PFM images over the same area have been taken with increasing temperature at the isothermal conditions. When temperature increases across the Néel temperature, the in-plane piezoelectric domain pattern changes largely indicating that the ferroelectric state is also altered and coupled to the accompanying magnetic transition. We have also observed that the clear double box poled state in the out-of-plane PFM images lasts even at high temperatures above the transition. Figure 6: Temperature-dependent PFM images of a T-BFO thin film. Three images (surface morphology at the left column, in-plane PFM at the middle column, out-of-plane PFM at the right column) have been taken simultaneously. The measurement sequence is from the top to the bottom, that is, increasing the temperature of the sample. Scale bars represent 1 μm. The PFM images were taken under amplitude contrast. Full size image Magnetoelectric susceptibility To understand the intriguing coupling between the ferroelectric and the magnetic orders in T-BFO, we have measured the transverse magnetoelectric susceptibility (MES) of the T-BFO as a function of external magnetic field at several selected temperatures ( Fig. 7 ). 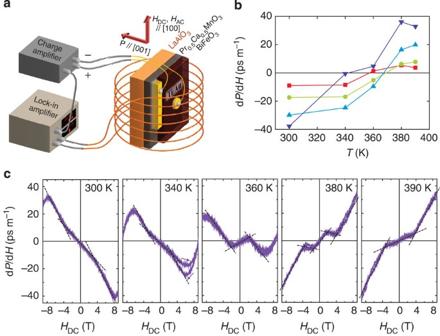Figure 7: Measurement of transverse magnetoelectric susceptibility of T-BFO. (a) Schematic illustration of the magnetoelectric susceptometer and the measurement configuration including the T-BFO film and the electrodes. Detailed measurement conditions are described at the Methods section. (b) Temperature-dependent MES values at several selected dc magnetic fields; 2 T (square symbols), 4 T (circle symbols), 6 T (triangle symbols pointing up) and 9 T (triangle symbols pointing down). These are extracted from isothermal field-sweep measurements shown inc. (c) Bias dc magnetic field dependence of MES of the T-BFO film measured from 300 to 390 K in a warming run. The sign of MES at a high-field region reverses as the sample passes across the transition temperature. The dashed guide lines indicate the slope change of MES. The schematic representation in Figure 7a shows the experimental setup of the MES measurement and the details are explained in Methods section. Taking into account that the pure T-BFO is in an anti-ferromagnetic state, we can get quite strong external field dependence of the MES. Also we have obtained totally different behaviour of the MES between the low-temperature and the high-temperature state as summarized in the Figure 7b,c . The MES below the transition temperature (300 K, 340 K) decreases roughly with a negative slope in external DC magnetic field sweep; whereas the high temperature one measured at 380 and 390 K shows overall tendency of positive slope. Several delicate slope changes have been detected as indicated by dashed lines in the Figure 7c . After the sample being cooled down, the negative slope observed at the 300 K was reproduced. Similar tendency has been also observed in another sample using an interdigital electrode geometry. Therefore, the MES measurement indicates that the nature of the spin-lattice coupling changes around the transition temperature. Whereas suppression of the MES around the transition temperature is most likely due to a cancelling effect inherited from phase coexistence or/and poly domain structure. More thorough experimental and theoretical studies are required to fully understand the magnetoelectric coupling of T-BFO. Figure 7: Measurement of transverse magnetoelectric susceptibility of T-BFO. ( a ) Schematic illustration of the magnetoelectric susceptometer and the measurement configuration including the T-BFO film and the electrodes. Detailed measurement conditions are described at the Methods section. ( b ) Temperature-dependent MES values at several selected dc magnetic fields; 2 T (square symbols), 4 T (circle symbols), 6 T (triangle symbols pointing up) and 9 T (triangle symbols pointing down). These are extracted from isothermal field-sweep measurements shown in c . ( c ) Bias dc magnetic field dependence of MES of the T-BFO film measured from 300 to 390 K in a warming run. The sign of MES at a high-field region reverses as the sample passes across the transition temperature. The dashed guide lines indicate the slope change of MES. Full size image As seen in the X-ray diffraction and PFM studies, it is clear that the magnetic transition is involved in the first-order structural transition where the ferroelectric state is altered too. Energy scales related to magnetic degrees of freedom are usually small; typically, it corresponds to the order of 1 K when a magnetic field of 1 T is applied. Thus, the concurrent transition seemingly has a structural origin. However, the magnetic order parameter decreases gradually with increasing temperature and vanishes at the transition temperature suggesting a second-order type of transition. We therefore have to reconcile the first-order structural/ferroelectric transition with the second-order-like magnetic transition. We cannot rule out the possibility that the magnetic ordering has a critical role to drive the transition. Similar first-order structural transition concurrent with the magnetic order has been observed in other compounds including a iron pnictide (BaFe 2 As 2 ) [38] and a layered perovskite ruthenate ((Sr,Ca) 2 RuO 4 ) [39] . However, these are not related to the ferroelectric order as is the case for the T-BFO. During the review process of this manuscript, we became aware of unpublished results regarding the magnetic transition temperature determined by Mössbauer spectroscopy [40] and by neutron scattering [41] . The neutron scattering data reveal somewhat lower T N ~324 K as compared with ours and the result of Mössbauer spectroscopy. This discrepancy is probably an indication of an ordering size effect, that is, the intensity of magnetic diffraction peaks may be relatively more suppressed as a result of finite size effect of magnetic domain in addition to decreasing magnitude of spin moments. We encourage more rigorous theoretical and experimental studies on spin-lattice interplay around the transition temperature. We present a room-temperature model system to deal with the interplay of magnetic and electric degrees of freedom by observing the concurrent antiferomagnetic and ferroelectric transition at the same temperature. This observation is thought provoking regarding the transition mechanism and potentially provides a pathway to magnetoelectric applications at room temperature. Moreover, our findings concerning the existence of the two different types of highly elongated BFO phases will stimulate more systematic investigations on the phase diagram of BFO as a function of strain and temperature. Growth of epitaxial films The epitaxial BFO thin films are grown using pulsed laser deposition. The KrF excimer laser with a wavelength of 248 nm with a repetition rate of 10 Hz was used. All films were grown on single crystal (001) LaAlO 3 substrates at a growth temperature of 650 °C and at an oxygen pressure of 100 mTorr. After finishing the growth, the films were cooled down to room temperature in oxygen environment at atmospheric pressure. The thickness of typical T-BFO films used was 30–40 nm. To get the R-BFO phase, we have grown very thick BFO (more than 250 nm in thickness) on the LaAlO 3 substrates so that they are relaxed and returned back to R-BFO. To prevent charging effects in measuring soft X-ray absorptions, a conducting LaNiO 3 layer with a few monolayers thickness was deposited underneath the BFO films. To fabricate capacitor structures for MES and to apply poling voltages in PFM measurements, we first grew epitaxially a conducting PCMO layer on LaAlO 3 substrates underneath the T-BFO film. Soft X-ray absorption spectroscopy The soft X-ray XAS measurements were carried out at beamline 2A at the Pohang Light Source, Pohang Accelerator Laboratory, and beamline 4.0.2 at the Advanced Light Source, Lawrence Berkeley National Laboratory. The measurements were performed in total electron yield (TEY) where the incident beam current and the sample drain current were simultaneously recorded to normalize the obtained spectrum with beam intensity. The polarization-dependent measurements were performed at the Fe L -edge and O K -edge without changing the measurement geometry for the R-BFO, T-BFO 1 films at Pohang Light Source. The sample temperature was controlled by using an open-circle cryostat with liquid nitrogen and in-vacuum resistive heater. After a temperature-dependent cycle from 100 to 500 K, we checked the XAS at 300 K and found no surface degradation caused by the heating. The sample normal direction was fixed at 70° to the photon propagation direction. The polarization-dependent XAS measurements at Fe L -edge were independently performed at various temperatures for the T-BFO 2 film in Advanced Light Source. The focus beam were incident on the sample at an angle of 75° from the sample normal direction; two electric polarizations, E//c and E//a, were selected by using the elliptically polarized undulator as presented in the inset of Figure 1a . X-ray diffraction Crystal structure was investigated using a X-ray diffractometer (Panalytical X'pert MRD Pro) with Cu K α1 radiation equipped with a high temperature oven (DHS-900) operating in an ambient environment. Each of the θ-2θ measurement took ~10 min after temperature stabilization of ~5 min. Analysis of reciprocal space maps The structural models of the T-BFO below and above T N are described in Supplementary Figure S3 and Supplementary Figure S4 , respectively. The highly elongated phases have large tetragonality ( c / a ~1.26) and thus it is often called tetragonal-like BFO. However, more careful structural analysis reveals peak splits in the reciprocal space maps indicating the real crystal symmetry should be lowered to a monoclinic unit cell rather than the tetragonal unit cell. To explain the observed peak splits in the reciprocal space maps, we have made a pesudocubic unit cell with a monoclinic tilt for the low temperature phase ( Supplementary Fig. S3a ). We introduce technical methods to extract the lattice parameters of the pseudocubic unit cell. The primitive vectors of the pseudocubic cell in real space and reciprocal space are presented in Cartesian coordinates ( Supplementary Fig. S3b ). The positions of {103} c and {113} c reflections in HL reciprocal space can be expected, as displayed in Supplementary Fig. S3c,d , which can be deduced on the basis of the reciprocal primitive vectors and fourfold twin structures around the normal [001] c . Similarly, a high-temperature structural model and expected reciprocal space maps are summarized in Supplementary Fig. S4 . These structural models of the low-temperature and the high-temperature phase correspond to the monoclinic unit cell represented by M C and M A [37] . It is worthwhile to mention that the high-temperature pseudocubic model is a special case of the M A , that is, the in-plane lattice parameter makes a square lattice. The tilt angle ( β ) stands for small deviation of the c -axis lattice vector from the exact normal and is related with the monoclinic angle using β =90− β H (90− β L ). Experimentally, the tilt angle ( β ) can be directly determined by the peak split in {103} c reflections for M C and by the peak split in {113} c reflections for M A . Capacitance and loss tangent measurement Interdigitated electrodes were made using thermal evaporation of Au through a patterned shadow mask on the T-BFO film (see the inset of Fig. 3a for the detailed dimension of the electrodes). The sample was installed in a Quantum design PPMS (physical property measurement system) (Quantum Design) equipped with LCR metre (Agilent E4980A, Agilent). An ac electric field with V ac ~2 V at the frequency of 100 kHz was employed for the measurement of the capacitance and the loss tangent. The temperature sweep rate was 4 K min −1 . PFM The PFM measurements were performed on a Digital Instruments Nanoscope-IV Multimode AFM equipped with external lock-in amplifiers. Using conductive AFM tips it is possible to measure local electrical and topographical properties both simultaneously and independently. The investigations were performed with commercially available TiPt-coated Si-tips (MikroMasch). Typical scan rates were 1.5 μm s −1 . All PFM images were taken in the mode of amplitude contrast where the signals correspond to real part ( X =amplitude times cos(phase)) of the PFM signal obtained through lock-in amplifiers. Magnetoelectric susceptibility measurement For MES d P /d H measurement, Ti/Au electrodes were deposited on top of T-BFO film surface (circular shape with a diameter of 50 μm) as well as the exposed PCMO surface (long bar shape). Gold wires were attached into the Ti/Au electrodes by use of a silver epoxy, which was then cured about 20 min at 90 °C. The sample is then mounted in a custom-made magnetoelectric susceptometer, in which a high-impedance charge amplifier and a lock-in amplifier are used for the phase-sensitive measurements of the modulated electric polarization by ac magnetic field generated by a solenoid (refer to Fig. 7a for schematic diagram of the instruments). The amplitude of the ac magnetic field was 4.18 Oe. By virtue of the phase-sensitive signal detection scheme, the magnetoelectric susceptometer could measure the modulation of charge as small as 10 −17 C at a frequency of 1 kHz. The samples were step by step warmed up from 300 to 390 K. Measurements were then performed in an isothermal condition at each temperature and the dc bias magnetic fields ( H DC ) was sequentially applied along the [100] direction from 0 to 9 to −9 to 0 T by use of a superconducting magnet in the PPMS (Quantum Design). How to cite this article: Ko, K.- T. et al . Concurrent transition of ferroelectric and magnetic ordering near room temperature. Nat. Commun. 2:567 doi: 10.1038/ncomms1576 (2011).